Luminescent proteins for high-speed single-cell and whole-body imaging The use of fluorescent proteins has revolutionized our understanding of biological processes. However, the requirement for external illumination precludes their universal application to the study of biological processes in all tissues. Although light can be created by chemiluminescence, light emission from existing chemiluminescent probes is too weak to use this imaging modality in situations when fluorescence cannot be used. Here we report the development of the brightest luminescent protein to date, Nano-lantern, which is a chimera of enhanced Renilla luciferase and Venus, a fluorescent protein with high bioluminescence resonance energy transfer efficiency. Nano-lantern allows real-time imaging of intracellular structures in living cells with spatial resolution equivalent to fluorescence and sensitive tumour detection in freely moving unshaved mice. We also create functional indicators based on Nano-lantern that can image Ca 2+ , cyclic adenosine monophosphate and adenosine 5′-triphosphate dynamics in environments where the use of fluorescent indicators is not feasible. These luminescent proteins allow visualization of biological phenomena at previously unseen single-cell, organ and whole-body level in animals and plants. Although fluorescence imaging is widely used, its dependence on external illumination prevents its universal application. For example, fluorescence imaging cannot be easily used to study light-dependent biological processes, such as visual photoreception or photosynthesis. Although optical recording of the light-sensitive retina has been successfully performed using 2-photon excitation with a 930-nm femtosecond laser [1] , this method is not versatile because many biological molecules have significant absorption at both visible and infrared wavelengths [2] . Therefore, methods based on fluorescence with both 1-photon and 2-photon excitation cannot always be used to study light-dependent biological processes. Moreover, fluorescence is incompatible with non-invasive deep tissue imaging of whole organisms and other applications where the cellular substrate is autofluorescent (for example, chloroplasts of photosynthetic plants), saturated with photopigments (porphyric hepatocytes, melanocytes or retinal pigment epithelia) or extremely photosensitive. Experimental problems also arise when external illumination is required, as for biological technologies such as optogenetics, chromophore-assisted light inactivation and photolysis of caged compounds, which prevents simultaneous use of fluorescence imaging. Finally, the general power density of external illumination for live-cell microscopy with fluorescence (sub W cm −2 ) sometimes causes phototoxic effects in visualized substrates, which alters cellular behaviour and ultimately leads to cell death. In contrast, chemiluminescence generates a visible light signal through a localized chemical reaction without the need for external illumination. Because the k cat values of conventional luciferases range from 0.1 for firefly luciferase (quantum yield=0.5) [3] to approximately 4.4 for Renilla luciferase (RLuc)8 (quantum yield=0.053) [4] , transient expression of micromolar concentrations of luciferases, for example, RLuc8, generates a power density of emitted light that is 1/10 3 that of the general power density required for fluorescence emission in live-cell imaging (approximately 0.1 μW cm −2 ). Therefore, although chemiluminescent proteins, including aequorin and luciferases, have been used to image living cells and organisms [5] , [6] , the light output from these proteins is insufficient to provide temporal and/or spatial resolution equivalent to fluorescence. In the case of luminous organisms, such as the sea pansy Renilla reniformis , the problem of low brightness has been solved in nature by the phenomenon of bioluminescence resonance energy transfer (BRET), in which the excited energy of a luminescent substrate, coelenterazine, bound to RLuc is efficiently transferred intermolecularly to the acceptor Renilla green fluorescent protein (quantum yield=0.3) by a Förster resonance energy transfer (FRET) mechanism, thereby increasing the emitted photon number approximately six-fold [7] . Based on this natural intermolecular BRET, intramolecular BRET probes, such as aequorin-GFP [8] and BAF-Y [9] , have been developed. Although these probes allow for live-cell imaging with improved resolution in space and time, they still underperform compared with fluorescent protein-based probes because of low brightness. To address this problem, we obtained a brighter RLuc by random mutagenesis and fusion to a yellow fluorescent protein (YFP) with high BRET efficiency. The fusion protein showed much brighter luminescence than BAF-Y, enabling not only real-time imaging of intracellular structures in living cells but also sensitive tumour detection in freely moving mouse. Moreover, we developed Ca 2+ , cyclic adenosine monophosphate (cAMP) and adenosine 5′-triphosphate (ATP) indicators based on this bright luminescent protein. These luminescent indicators will allow visualization after the optical control of cellular or enzymatic activity at the single-cell, organ and whole-body level in animals and plants. Design and application of the bright luminescent protein To improve brightness, we designed a chimeric protein based on eBAF-Y [9] ( Supplementary Note 1 ), which is a fusion of enhanced YFP and an enhanced RLuc, RLuc8 ( [4] ). Because BRET efficiency, and thus brightness, depends on the photochemical and physical properties of the donor and acceptor, we honed these parameters by improving donor brightness, maximizing spectral overlap between the donor emission and acceptor absorbance using Venus [10] and optimizing the spatial arrangement of the donor and acceptor in the fusion construct ( Supplementary Note 1 , Supplementary Fig. S1 and Supplementary Table S1 ). The resulting protein, which we called Nano-lantern, reminiscent of a light source with nanometre scale ( Fig. 1a ), exhibited 5.3 and 2.9 times greater luminescence than RLuc8 and eBAF-Y, respectively, over the entire emission range ( Fig. 1b ). The improved brightness of Nano-lantern should generate power densities in the range of 1 μW cm −2 (versus 0.1 μW cm −2 for RLuc8) following transient overexpression in the micromolar range in human cells, and thus increase imaging potential. 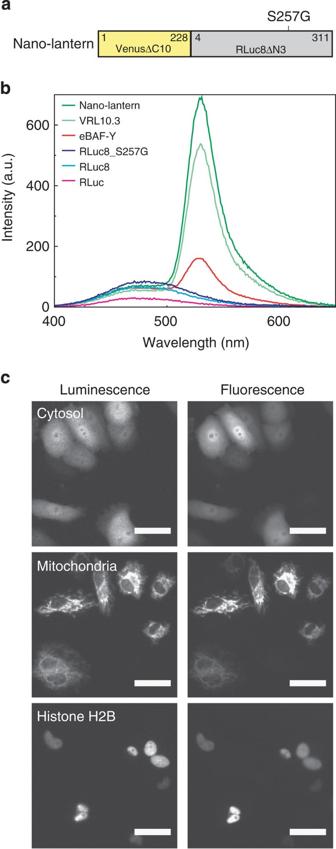Figure 1: Development of the bright luminescent protein Nano-lantern. (a) Schematic of the domain structure of Nano-lantern. Numbers represent the relative amino-acid position in the original protein. (b) Emission spectra of equimolar amounts of the luminescent proteins Nano-lantern, VRL10.3, eBAF-Y9, RLuc8_S257G, RLuc8 and RLuc. Emission spectra measurements were performed at least in triplicate, and the averaged data are shown. (c) Luminescence (left) and fluorescence (right) imaging of HeLa cells expressing Nano-lantern targeted to cytoplasm, mitochondria and histone H2B. The exposure times for the luminescence images were 3 s, 3 s and 1 s, respectively. The exposure time for all fluorescence images was 1 s. The reference fluorescence signal was captured by exciting Venus with light at 490 nm. Scale bars, 50 μm. Figure 1: Development of the bright luminescent protein Nano-lantern. ( a ) Schematic of the domain structure of Nano-lantern. Numbers represent the relative amino-acid position in the original protein. ( b ) Emission spectra of equimolar amounts of the luminescent proteins Nano-lantern, VRL10.3, eBAF-Y 9 , RLuc8_S257G, RLuc8 and RLuc. Emission spectra measurements were performed at least in triplicate, and the averaged data are shown. ( c ) Luminescence (left) and fluorescence (right) imaging of HeLa cells expressing Nano-lantern targeted to cytoplasm, mitochondria and histone H2B. The exposure times for the luminescence images were 3 s, 3 s and 1 s, respectively. The exposure time for all fluorescence images was 1 s. The reference fluorescence signal was captured by exciting Venus with light at 490 nm. Scale bars, 50 μm. Full size image Indeed, when Nano-lantern was expressed in HeLa cells, a luminescence image with quality almost comparable to that of fluorescence images was obtained. Nano-lantern and fusions with defined localization tags enabled visualization of cell compartments and organelles, such as the cytoplasm, mitochondria and nucleus (histone H2B), in living cells by using low magnification lens (X20 dry objective) with brief, 1–3-s exposures ( Fig. 1c ). Nano-lantern also allowed for visualization of finer structures, including microfilaments, microtubules and their tips (EB3) with a high magnification lens (X60 oil-immersion objective) and longer, 3–60 s, exposures ( Supplementary Fig. S2 ). Therefore, the enhanced luminescent signal (μW cm −2 ) from Nano-lantern enables imaging at high spatial resolution until at least the subcellular level, with a quality approaching that of fluorescent protein (FP)-based imaging. This is because although the power density of the emitted light of Nano-lantern is still ~1/10 2 smaller than that of general fluorescence emissions (at ~100 μW cm −2 ), image quality is defined by the signal-to-noise ratio (S/N ratio). In fluorescence imaging, this is compromized by high noise levels from stray excitation light and autofluorescence from both the sample and the medium. In chemiluminescence imaging, quality does not suffer from low signal levels because of the very low noise level. Because external illumination is not needed, an adequate S/N ratio is preserved. Currently, chemiluminescence is commonly used for non-invasive tumour detection in living mice for tumour metastasis research and anti-cancer-drug screening [11] . Brighter luminescence should enable detection of smaller tumours. Indeed, when adenocarcinoma colon26 cell lines that stably express Nano-lantern or RLuc8 (colon26/Nano-lantern and colon26/RLuc8) was subcutaneously implanted into BALB/c nude mice ( Fig. 2a ), and we detected as few as 10 3 Nano-lantern-expressing cells 1 day after transplantation ( Fig. 2b ), which is 1 order of magnitude better than RLuc8-expressing tumours ( Fig. 2c ). 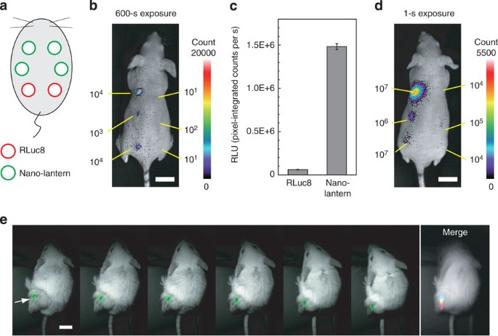Figure 2: Luminescence imaging of mice with Nano-lantern-expressing tumours. (a) Position of colon26 cells expressing Nano-lantern (green circles) or RLuc8 (red circles) in the transplanted mice (dorsal view). (b,d) Representative luminescence images of the indicated numbers of injected cells at 600 s (b) and 1 s exposures (d). (c) Comparison in relative light units (RLU, pixel-integrated counts per s) of 1 × 107cells of colon26/RLuc8 and Nano-lantern. Measurements were performed in triplicate, and the averaged data and s.d. are shown. (e) Consecutive frames of video-rate images of Nano-lantern-expressing tumour cells in an unshaved mouse. The luminescent signal every 60 ms is shown in green in the still images and as a series of pseudo colours (blue, cyan, green, yellow, red and magenta) in the merged image. Scale bars, 1 cm. Figure 2: Luminescence imaging of mice with Nano-lantern-expressing tumours. ( a ) Position of colon26 cells expressing Nano-lantern (green circles) or RLuc8 (red circles) in the transplanted mice (dorsal view). ( b , d ) Representative luminescence images of the indicated numbers of injected cells at 600 s ( b ) and 1 s exposures ( d ). ( c ) Comparison in relative light units (RLU, pixel-integrated counts per s) of 1 × 10 7 cells of colon26/RLuc8 and Nano-lantern. Measurements were performed in triplicate, and the averaged data and s.d. are shown. ( e ) Consecutive frames of video-rate images of Nano-lantern-expressing tumour cells in an unshaved mouse. The luminescent signal every 60 ms is shown in green in the still images and as a series of pseudo colours (blue, cyan, green, yellow, red and magenta) in the merged image. Scale bars, 1 cm. Full size image The increased brightness of Nano-lantern allowed for imaging of 10 5 and 10 6 cells at 0.1 and 1 Hz sampling rates, respectively ( Fig. 2d ). Surprisingly, we could even obtain video rate (30 Hz) imaging of tumours 17 day after implantation of 10 6 of tumour cells in freely moving unshaved mice ( Fig. 2e and Supplementary Movie 1 ). In previous reports of luminescent tumour cell imaging in non-anaesthetized mice [12] , successful images were only obtained with nude mice, larger tumour samples and prolonged exposure times (160 or 200 versus 33 ms in this report). Increased sensitivity and faster imaging without the need for anaesthesia using Nano-lantern greatly facilitates the analysis of tumour growth and metastasis in living animals. Functional indicators based on Nano-lantern Having demonstrated the benefit of the improved luminescent properties of Nano-lantern, micrometre spatial resolution in living cells and improved tumour resolution in whole animals, we sought to develop functional indicators for bioactive molecules such as Ca 2+ , cAMP and ATP based on Nano-lantern. Thus far, two types of chemiluminescence-based functional indictors have been reported; one uses the complementation of split luciferase (CSL), in which the luciferase molecule is split, with one portion fused to the sensor domain of a bioactive molecule and the other to a peptide that binds the sensor domain. This type of indicator emits a signal upon bioactive molecule-binding-mediated reconstitution of the split luciferase [13] . The other uses a BRET-based indicator composed of the sensor domain of a bioactive molecule flanked by an intact chemiluminescent donor and a fluorescent acceptor, in this case, a cellular response is detected as a change in BRET efficiency [14] . Although CSL-type indicators have a larger signal change, their absolute intensity is often too low to be imaged. Conversely, BRET-based type indicators have sufficient signal intensity for imaging; however, its signal change upon target molecule binding is generally small. To overcome these drawbacks, we sought to insert a sensor domain into Nano-lantern to create a hybrid CSL/BRET indicator that would exhibit a signal change with sufficient intensity for imaging ( Supplementary Fig. S3a ). A Ca 2+ indicator based on Nano-lantern Given the novel hybrid approach, we first sought to develop a Nano-lantern-based indicator for Ca 2+ , one of the most important second messengers in living cells. We cloned the Ca 2+ -sensing domain (CaM-M13) of yellow cameleon, an established FRET-based Ca 2+ -indicator [15] , and searched for the optimal insertion site in Nano-lantern that would yield a large signal change and preserve high intensity emission. Other important properties, including Ca 2+ affinity and reversibility of the catalytic activity of luciferase, were also examined. Ultimately, of the sites tested, we found that insertions into the non-structural Gly 228 /Gly 229 loop in RLuc8 that links the hydrolase and cap domains were well tolerated ( Supplementary Fig. S3b and Supplementary Note 2 ). The resulting construct, named Nano-lantern (Ca 2+ ), showed a 300% signal change at 35% brightness of the parental protein at saturating Ca 2+ concentrations ( Fig. 3a ). The Ca 2+ affinities of Nano-lantern (Ca 2+ ) and its derivatives ( Supplementary Fig. S4 and Supplementary Table S2 ) were almost identical to that of the parental yellow cameleon series, suggesting that reconstitution of split-Rluc8 in Nano-lantern (Ca 2+ ) did not interfere with the Ca 2+ -induced conformational change in the CaM-M13 domain ( Supplementary Note 2 ). 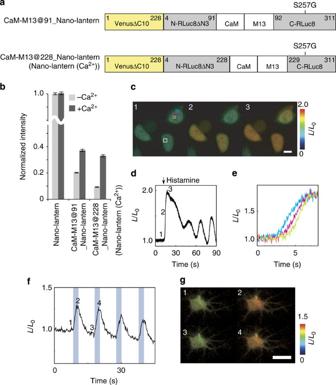Figure 3: Development of a Nano-lantern-based luminescent Ca2+indicator. (a) Schematic representation of the domain structures of CaM-M13@91_Nano-lantern and CaM-M13@228_Nano-lantern (Nano-lantern (Ca2+)). (b) Relative brightness of recombinant Nano-lantern, CaM-M13@91_Nano-lantern and CaM-M13@228_Nano-lantern (Nano-lantern (Ca2+)), with or without Ca2+. Measurements were performed at least in triplicate, and the averaged data and s.d. are shown. (c) A series of pseudo-coloured ratio images of HeLa cells expressing Nano-lantern (Ca2+) taken at video rate, following histamine stimulation. Scale bar, 10 μm. (d) Time course of theL/L0ratio change at an ROI (white box in (c)) in a HeLa cell expressing Nano-lantern (Ca2+). Number indicates the time point of each image in (c). Representative data from at least five experiments are shown in (d) and (e). (e) A typical time course of the spatialL/L0ratio change in ROIs (cyan, magenta and yellow boxes in (c)) in another HeLa cell. (f) Time course of theL/L0ratio change in a rat hippocampal neuron co-expressing Nano-lantern (Ca2+) with the ChR2. ChR2 was repeatedly photo-activated in illumination sessions (~2 s), consisting of 15 cycles of camera exposure (100 ms) and pulses of blue light (0.8 ms) that were delivered during periods (30 ms) when camera exposure was off. Numbers indicate the time points of each image in (g). Representative data from five measurements are shown. (g) A series of pseudo-coloured ratio images of a rat hippocampal neuron expressing Nano-lantern (Ca2+). Scale bar, 10 μm. Figure 3: Development of a Nano-lantern-based luminescent Ca 2+ indicator. ( a ) Schematic representation of the domain structures of CaM-M13@91_Nano-lantern and CaM-M13@228_Nano-lantern (Nano-lantern (Ca 2+ )). ( b ) Relative brightness of recombinant Nano-lantern, CaM-M13@91_Nano-lantern and CaM-M13@228_Nano-lantern (Nano-lantern (Ca 2+ )), with or without Ca 2+ . Measurements were performed at least in triplicate, and the averaged data and s.d. are shown. ( c ) A series of pseudo-coloured ratio images of HeLa cells expressing Nano-lantern (Ca 2+ ) taken at video rate, following histamine stimulation. Scale bar, 10 μm. ( d ) Time course of the L / L 0 ratio change at an ROI (white box in ( c )) in a HeLa cell expressing Nano-lantern (Ca 2+ ). Number indicates the time point of each image in ( c ). Representative data from at least five experiments are shown in ( d ) and ( e ). ( e ) A typical time course of the spatial L / L 0 ratio change in ROIs (cyan, magenta and yellow boxes in ( c )) in another HeLa cell. ( f ) Time course of the L / L 0 ratio change in a rat hippocampal neuron co-expressing Nano-lantern (Ca 2+ ) with the ChR2. ChR2 was repeatedly photo-activated in illumination sessions (~2 s), consisting of 15 cycles of camera exposure (100 ms) and pulses of blue light (0.8 ms) that were delivered during periods (30 ms) when camera exposure was off. Numbers indicate the time points of each image in ( g ). Representative data from five measurements are shown. ( g ) A series of pseudo-coloured ratio images of a rat hippocampal neuron expressing Nano-lantern (Ca 2+ ). Scale bar, 10 μm. Full size image To compare the performance of this Ca 2+ indicator to a known standard, we expressed Nano-lantern (Ca 2+ ) in HeLa cells. Following stimulation with 10 μM histamine, an acute Ca 2+ spike (S/N=70) followed by Ca 2+ oscillations with smaller amplitudes (S/N=29) were detected with a sampling rate as fast as 30 Hz ( Fig. 3c ). We could even observe the propagation of a cytoplasmic Ca 2+ wave from one end of the cell to the other, as was previously observed using yellow cameleon [15] ( Fig. 3e and Supplementary Movie 2 ). Histamine-induced Ca 2+ oscillations were abolished by the addition of the histamine receptor antagonist cyproheptadine, confirming that the luminescent signal change reflects changes in cytoplasmic [Ca 2+ ] ( Supplementary Fig. S5 ). Previous CSL-based Ca 2+ indicators [13] were not fully reversible in response to physiological or stimulated Ca 2+ release. We confirmed by co-imaging Nano-lantern (Ca 2+ ) with R-GECO1 [16] that the kinetics of Nano-lantern (Ca 2+ ) parallel those of fluorescence-based probes ( Supplementary Fig. S6 ). Encouragingly, Nano-lantern (Ca 2+ ), when expressed in dissociated rat hippocampal neurons ( Supplementary Fig. S7 ), and imaged at 10 Hz, could report spontaneous cytoplasmic [Ca 2+ ] spikes and transient [Ca 2+ ] changes due to reversible stimulation (50 mM KCl). To realize the theoretical advantage of Ca 2+ imaging using luminescence probes over fluorescence-based indicators, we performed Ca 2+ imaging combined with the control of neuronal activity using optogenetic tools. Ectopic expression of photoreceptor proteins, such as halorhodopsin and channelrhodopsin2 (ChR2), has enabled the functional analysis of neuronal cells and their networks with ms time resolution [17] . Yet, these tools are spectrally incompatible with fluorescent Ca 2+ indicators. Excitation light can be used either to control the photoreceptor or to measure the Ca 2+ transient, but not for both in the same cell at the same time. Because luminescence imaging can be performed in the absence of external light, it can be partnered with an optogenetic strategy without undesired interference due to the activity of the photoreceptor. To demonstrate this, we co-expressed Nano-lantern (Ca 2+ ) and ChR2 in dissociated rat hippocampal neurons. The luminescent signal was imaged every 100 ms, and ChR2 was activated with a 0.8-ms pulse of blue light (438 nm) during the dead time of the CCD chip for data transfer [18] . In response to 15 cycles of activation light, a rapid increase was observed in the luminescent signal ( Fig. 3f and Supplementary Movie 3 ). We also detected a gradual decrease in the signal to the basal level when the illumination was terminated. Catalytic consumption of substrate (coelenterazine-h) causes a gradual decrease in both the baseline and the amplitude of transients. These results suggest that these synergistic neurobiology tools can now be combined into a single experimental approach. In the future, it may also be possible to combine other optical control systems, such as chromophore-assisted light inactivation of target molecules [19] and photolysis of caged compounds [20] , with luminescent functional indicators. Improved cAMP indicators based on Nano-lantern Imaging intracellular cAMP, another important second messenger, using fluorescent indicators has been challenging because of the small signal change (1–15%) with current FP-based indicators [21] , [22] , [23] . To examine whether the CSL/BRET hybrid strategy could be applied to construct a high-performance cAMP indicator, we cloned a series of cAMP-binding motifs from the PKA regulatory subunit or EPAC1, into Nano-lantern at the 228/229 position (similar to in Nano-lantern (Ca 2+ )) ( Supplementary Fig. S8a ). Recombinant proteins were purified and screened for intensity changes in response to cAMP. Among the nine constructs tested, three cAMP-recognition motifs gave a large signal change with distinct cAMP affinities ( K d =0.4, 1.6 and 3.3 μM), and one of these three, Nano-lantern containing a fragment of EPAC1 (G170 to A327 with Q270E), which we named Nano-lantern (cAMP1.6) (from its K d ), showed the largest signal increase (130%) upon cAMP stimulation ( Fig. 4a , Supplementary Fig. S8b–d and Supplementary Note 3 ). In contrast, FRET-based indicators with an identical cAMP-recognition domain showed only a small signal change (11.7% for CFP/YFP-based constructs; Supplementary Fig. S8e and Supplementary Note 3 ). 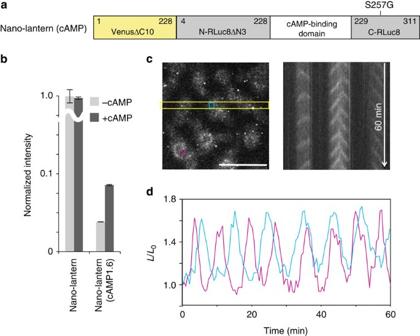Figure 4: Development of a Nano-lantern-based luminescent cAMP indicator. (a) Schematic of the domain structure of Nano-lantern (cAMP). (b) Relative brightness of recombinant Nano-lantern and Nano-lantern (cAMP) with or without cAMP. These measurements were performed at least in triplicate, and the averaged data and s.d. are shown. (c) A cAMP image of ~100,000D. discoideumcells expressing Nano-lantern (cAMP1.6) during aggregative morphogenesis. Scale bar, 1 mm. (d) Space and time plot along the yellow lines shown in (c) for 60 min. (e) Time course of the luminescence intensity change at the ROIs indicated in (c). These are typical data from five measurements. Figure 4: Development of a Nano-lantern-based luminescent cAMP indicator. ( a ) Schematic of the domain structure of Nano-lantern (cAMP). ( b ) Relative brightness of recombinant Nano-lantern and Nano-lantern (cAMP) with or without cAMP. These measurements were performed at least in triplicate, and the averaged data and s.d. are shown. ( c ) A cAMP image of ~100,000 D. discoideum cells expressing Nano-lantern (cAMP1.6) during aggregative morphogenesis. Scale bar, 1 mm. ( d ) Space and time plot along the yellow lines shown in ( c ) for 60 min. ( e ) Time course of the luminescence intensity change at the ROIs indicated in ( c ). These are typical data from five measurements. Full size image To examine the ability of Nano-lantern (cAMP1.6) to detect intracellular cAMP concentration changes, we used Dictyostelium discoideum cells because cytoplasmic cAMP concentration (hereafter [cAMP]) in Dictyostelium cells increases in response to extracellular cAMP stimulation [24] , [25] , which indirectly increases [cAMP] through the action of the cell-surface receptor and cAMP synthase (adenylate cyclase A). Cells stably expressing Nano-lantern (cAMP1.6) whose K d was best fitted to the estimated range of oscillating cellular [cAMP] ( Supplementary Fig. S8d and Supplementary Table S3 ) [26] showed a rapid increase in luminescent signal (40% increase in initial intensity), followed by a gradual decay in response to 100 μM cAMP stimulation ( Supplementary Fig. S9 ). These luminescence signal changes do indeed reflect cytoplasmic cAMP dynamics, as we confirmed that this transient cAMP-stimulated signal increase was lost in adenylate cyclase A mutant cells ( Supplementary Fig. S10 ). During morphogenesis, populations of Dictyostelium cells form circular and spiral aggregation patterns [27] . This is achieved by the repeated intracellular synthesis and intercellular relay of cAMP (at a 6–10-min interval), which functions as a chemoattractant molecule. Direct imaging of this with fluorescence reporters has never been previously possible because of their limited dynamic range. When cells stably expressing Nano-lantern (cAMP1.6) were cultured on an agar plate (10 6 cells cm −2 ), we observed a propagating spiral wave of cAMP with a 6-min periodicity that had a larger signal change ( Fig. 4c , and Supplementary Movie 4 ) than that detected with a currently available FRET-based indicator ( Supplementary Fig. S11 and Supplementary Movie 5 ). We were able to successfully detect cAMP at the single-cell level in Dictyostelium amoebae (cell volume, approximately 1/20 that of HeLa cells) with FRET-based indicators ( Supplementary Fig. S11b ); however, this was not possible with Nano-lantern (cAMP). In fact, approximately 20 single cells were required to obtain a luminescence image at high magnification ( Supplementary Fig. S9 ) due to the low absolute intensity in this organism because of its lower expression compared with that in mammalian cells. However, these results still demonstrate that luminescent indicators have a clear performance advantage over fluorescence-based indicators when performing macroscopic analysis of populations of living cells for prolonged periods without obvious cell injury. Visualizing ATP production in plant chloroplasts Luminescence imaging can be applied in systems where fluorescence observation is impossible. A typical example is the chloroplast of photosynthetic plants, which converts the energy of sunlight into chemical energy in the form of NADPH and ATP. Fluorescence-based imaging cannot provide the needed spatiotemporal resolution for this process due to the strong autofluorescence of chlorophyll and the intrinsic photosensitivity of photosynthesis. Therefore, as another demonstration of luminescence-based functional imaging, we sought to visualize the dynamics of ATP production and utilization in chloroplasts. To this end, we developed a Nano-lantern-based ATP indicator using the ε subunit of the bacterial F o F 1 -ATP synthase similar to that found in the fluorescent ATP indicator ATeam [28] . This was also inserted into the 228–229 position in a modified Nano-lantern (VRL10.0_S257G) ( Supplementary Note 4 ). The generated construct, which we named Nano-lantern (ATP1), exhibited a 200% increase in light output upon the addition of ATP with a K d of 0.3 mM ( Fig. 5a , Supplementary Fig. S12 and Supplementary Table S4 ). 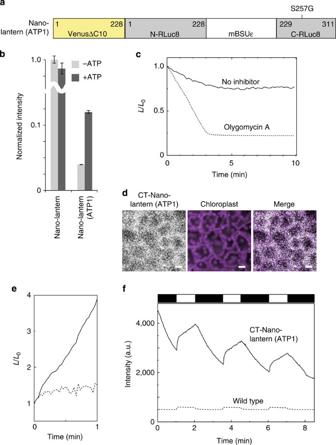Figure 5: Development of a Nano-lantern-based luminescent ATP indicator. (a) Schematic of the domain structure of Nano-lantern (ATP1). (b) Relative brightness of recombinant Nano-lantern and Nano-lantern (ATP1) with or without ATP. These measurements were performed at least in triplicate, and the averaged data and s.d. are shown. (c) Time course of the luminescence intensity change in a plant leaf expressing Nano-lantern (ATP1) with (dashed line) or without (solid line) the mitochondrial ATP synthesis inhibitor oligomycin A. Representative data from five measurements are shown. (d) Plant leaf luminescence images of CT-Nano-lantern (ATP1), chloroplast autofluorescence and merge. Scale bar, 20 μm. (e) A typical pattern of the time course of the luminescence intensity change in a plant leaf expressing CT-Nano-lantern (ATP1) with (dashed line) or without (solid line) the photosynthesis inhibitor 3-(3,4-dichlorophenyl)-1,1-dimethylurea with weak light irradiation (0.3 mW cm−2). Representative data from five measurements are shown. (f) A typical pattern of the time course of the luminescence intensity change in a plant leaf expressing CT-Nano-lantern (ATP1) (solid line) or in a wild-type plant (dashed line) with pulsed light (8.2 mW cm−2) indicated as a white rectangle in the scheme above the graph. Representative data from five measurements are shown. Figure 5: Development of a Nano-lantern-based luminescent ATP indicator. ( a ) Schematic of the domain structure of Nano-lantern (ATP1). ( b ) Relative brightness of recombinant Nano-lantern and Nano-lantern (ATP1) with or without ATP. These measurements were performed at least in triplicate, and the averaged data and s.d. are shown. ( c ) Time course of the luminescence intensity change in a plant leaf expressing Nano-lantern (ATP1) with (dashed line) or without (solid line) the mitochondrial ATP synthesis inhibitor oligomycin A. Representative data from five measurements are shown. ( d ) Plant leaf luminescence images of CT-Nano-lantern (ATP1), chloroplast autofluorescence and merge. Scale bar, 20 μm. ( e ) A typical pattern of the time course of the luminescence intensity change in a plant leaf expressing CT-Nano-lantern (ATP1) with (dashed line) or without (solid line) the photosynthesis inhibitor 3-(3,4-dichlorophenyl)-1,1-dimethylurea with weak light irradiation (0.3 mW cm −2 ). Representative data from five measurements are shown. ( f ) A typical pattern of the time course of the luminescence intensity change in a plant leaf expressing CT-Nano-lantern (ATP1) (solid line) or in a wild-type plant (dashed line) with pulsed light (8.2 mW cm −2 ) indicated as a white rectangle in the scheme above the graph. Representative data from five measurements are shown. Full size image When expressed in a live plant leaf, Nano-lantern (ATP1) was able to detect the decrease in cytoplasmic ATP levels resulting from the addition of a mitochondrial ATP synthase inhibitor, oligomycin A ( Fig. 5c ). To visualize ATP production in chloroplasts during photosynthesis, transgenic Arabidopsis plants were constructed that could target Nano-lantern (ATP1) to the chloroplast stroma by using a transit peptide fusion [29] (CT-Nano-lantern (ATP1)). The luminescent signal for CT-Nano-lantern (ATP1) in the mesophyll of leaf cells overlapped with the red autofluorescence signal of the chloroplasts ( Fig. 5d ), and an increase in ATP levels was detected after weak light irradiation. This response was effectively suppressed by treatment with the photosynthesis inhibitor, 3-(3,4-dichlorophenyl)-1,1-dimethylurea [30] ( Fig. 5e ), demonstrating that this response in ATP levels was photosynthesis dependent. Further monitoring of the regulation of chloroplast ATP levels was possible by pulsing strong photo-irradiation ( Fig. 5f and Supplementary Movie 6 ). During photo-irradiation, ATP levels increased rapidly in the first few seconds, and then continued to increase at a moderate rate. We speculate that this slower increase is due to downregulation of the photosynthesis rate by energy-dependent quenching (qE quenching) [31] , a rapid mechanism used to modulate the amount of light accepted and to prevent the harmful effects of excess light irradiation. To our knowledge, this is the first visualization of qE quenching-mediated downregulation of ATP synthesis in live plant cells. Taken together, these results demonstrate the potential of Nano-lantern-based indicators as powerful tools for functional observation in biological materials with strong autofluorescence and photosensitivity. Other cells with these properties include porphyric hepatocytes and erythrocytes, which accumulate the photo-sensitizing substance porphyrin, and retinal ganglion cells, which absorb light in animal retinas. Nano-lantern-based indicators may be useful for analysing the native properties of these cells, which cannot always be determined with existing FP (because of the need for external illumination) or chemiluminescent indicators (because of their poor indicator performance). By optimizing the BRET efficiency between Venus and improved RLuc8, we developed Nano-lantern, the brightest luminescent protein reported to date. This enhanced brightness enables luminescent imaging on a micrometre scale in single cells, and tumour imaging in freely moving, unshaved animals. We expect that the increased brightness of Nano-lantern will make more advanced applications possible, such as high-throughput drug screening and single-cell tracking in living animals and plants. In addition, Nano-lantern can help realize the other advantages of low-intensity light imaging, including diminished photobleaching and phototoxicity, which allow for prolonged observation without harming the cellular substrate. However, rapid consumption of the luminescent substrate by Nano-lantern hampers prolonged observation of biological events, especially, in the case of whole-body imaging. Therefore, to facilitate indefinite observation, a method that is applicable to the entire organism and provides a continuous luminescent substrate must be developed. An important aspect of this study is the development of a simple method for the construction of high-performance luminescence-based indicators by inserting the sensor domain of bioactive molecules into the non-structural Gly 228 /Gly 229 loop of the RLuc8 moiety in Nano-lantern. However, saturation screening to determine better insertion sites might also improve the functional indicator performance in terms of the rate constants for the association and dissociation of the ligand with the indicator, both of which are important properties for reliable reporting of bioactive molecule dynamics. Finally, a further increase in brightness is clearly desirable. The efficiency of intermolecular BRET between RLuc and Renilla green fluorescent protein was reported to be 1.0 (ref. 7 ), suggesting that Nano-lantern, the BRET efficiency of which is estimated to be approximately 0.2, could be improved. If this was achieved, luminescent proteins might allow imaging on even smaller spatial or temporal scales, possibly even at the single-molecule level. General The detailed experimental conditions are described in the Supplementary Methods and Supplementary Tables S5–S7 . Screening of bright RLuc8 gene libraries RLuc8 cDNA was generated by introducing eight mutations, A55T/C124A/S130A/K136R/A143M/M185V/M253L/S287L, into pGL4.70 [hRLuc] (Promega) by site-directed mutagenesis [4] . To obtain the cDNA libraries of mutated RLuc8 (mut-RLuc8), 30 rounds of error-prone PCR were performed under conditions to achieve a mutation rate of 5-bp/kb. Escherichia coli JM109 (DE3) cells were transformed with pRSET B _mut-RLuc8 and were spread on LB/ampicillin agar plates. Following a 20-h incubation at 37 °C, the E. coli colonies were sprayed with a phosphate-buffered saline (PBS) solution containing 5 μg ml −1 coelenterazine-h and were examined with an LAS-1000 luminescence imaging system (GE Healthcare). The brightest colonies were picked, and their brightness was tested. Construction of Nano-lantern To obtain eBAF-Y [9] cDNA, the enhanced YFP and RLuc8 regions were amplified by PCR. The two resulting fragments were ligated into the pRSET B vector (Life Technologies) to generate pRSET B _eBAF-Y. Venus, the circularly permutated Venus series (cp50, 157, 173, 195 and 229Venus) [15] , and the C-terminally 10 amino-acid-truncated Venus (VenusΔC10) were amplified by PCR. RLuc8 and the N-terminally 1–6-truncated RLuc8 (ΔN1–6) were amplified by PCR. The resulting fragments of Venus and RLuc were ligated into the BamH I/ EcoR I site of the pRSET B vector to yield a series of pRSET B _Venus-RLuc8 fusion proteins. Construction of Nano-lantern (Ca 2+ ) To insert a Ca 2+ -sensing domain into the RLuc8 moiety of Nano-lantern, a cDNA fragment encoding the CaM-M13 peptide of YC3.60 [15] was amplified by PCR to add Nco I and Sac I sites to its 5′ and 3′ ends by using the fCaM ( Nco I) and rM13 ( Sac I) primers, respectively. These restriction sites were also introduced at the 91/92 or 228/229 position of RLuc8_S257G in pRSET B _RLuc8_S257G and pRSET B _Nano-lantern by PCR. These fragments were then ligated to yield pRSET B _CaM-M13@91_RLuc8_S257G, pRSET B _CaM-M13@91_Nano-lantern and pRSET B _CaM-M13@228_Nano-lantern. Construction of Nano-lantern (cAMP) The cDNA clone encoding the human PKA regulatory subunit Iα was purchased from DNAFORM (Japan), and the cDNA fragments corresponding to the cAMP-binding domain and its flanking region and Nano-lantern region were amplified by PCR. The obtained fragments were ligated to yield pRSET B _Nano-lantern (cAMP). A Q270E mutation was introduced into EPAC1 by site-directed mutagenesis. A fragment encoding the 12-amino-acid linker PWNWDSGCSREG was attached to the junction between 228 of Nano-lantern and the N-terminus of the cAMP-binding motif by inserting an oligonucleotide cassette. Construction of Nano-lantern (ATP) The cDNA fragment encoding the ATP-recognition domain (the ε subunit of the bacterial F o F 1 -ATP synthase) was PCR-amplified using ATeam1.03 cDNA as a template [28] . The Nco I_CaM-M13_ Sac I fragment of Nano-lantern (Ca 2+ ) was replaced with the ATP-recognition motif to yield pRSET B _Nano-lantern (ATP0). RLuc8_S257G (ΔN3) of pRSET B _Nano-lantern (ATP0) was replaced with RLuc8_S257G (ΔN0) to generate pRSET B _Nano-lantern (ATP1). Protein purification and in vitro spectroscopy E. coli strain JM109 (DE3) was transformed with a pRSET B vector carrying Nano-lantern and its derivative cDNA and was grown at 23 °C. Recombinant proteins were purified using Ni-NTA agarose (Qiagen) and then diluted to 20 nM in 50 mM HEPES (pH 7.2). The emission spectra of the purified proteins were measured using a micro-plate reader (SH-9000; Corona Electric) or a spectrofluorometer (F-4500; Hitachi). A final concentration of 1–10 μM coelenterazine-h was used as the luminescent substrate for these measurements. Experiments were performed at least in triplicate, and the averaged data were used for further analysis. For Nano-lantern (cAMP), × 6 His-tagged recombinant Nano-lantern (cAMP) proteins were expressed in Dictyostelium cells and purified using Ni-NTA agarose, because synthetic genes containing cAMP-recognition motifs were not efficiently expressed in E. coli . The emission spectrum of 100 nM Nano-lantern (cAMP) was measured in the presence of 6 μM coelenterazine-h using a spectrophotometer (F-4500; Hitachi). For the FRET constructs, 200 μM recombinant protein was used in the spectral analysis. The emission spectrum upon excitation with 425 nm light was measured in the presence or absence of 100 μM cAMP. Preparation and imaging of mice All animal experiments were carried out in accordance with the Principles of Laboratory Animal Care, as adopted and promulgated by the Guidelines for Animal Experiments at Kyoto University and Hokkaido University. For tumour cell imaging, 5-week-old male nude BALB/c mice ( nu/nu ) were anesthetized. At six different sites on the back, 1 × 10 1 –1 × 10 7 colon26 cells expressing RLuc8 or Nano-lantern were subcutaneously transplanted, as illustrated in Fig. 2a . On the next day, the mice were anesthetized again, and 80 μg of coelenterazine-h/mouse in 20% ethanol: 80% PBS (in a final volume of 200 μl) was intravenously administered. For the video-rate imaging of freely moving mice, 1 × 10 6 colon26 cells stably expressing Nano-lantern were subcutaneously implanted into the back of anesthetized 5-week-old male BALB/c mice. On the 17th day after implantation, 8 μg of coelenterazine-h/mouse in 20% ethanol: 80% PBS (in a final volume of 60 μl) was injected into the tumour. Detailed imaging conditions are described in Supplementary Methods and Supplementary Table S6 . Preparation and imaging of rat hippocampal neuron cultures On day in vitro 7, dissociated rat hippocampal neurons cells were transfected with pcDNA3_ Nano-lantern (Ca 2+ ) and pcDNA3.1_hChR2 by calcium phosphate precipitation. The neuronal cells were imaged on day in vitro 9–11 by using an inverted wide-field epifluorescence microscope as described in Supplementary Methods . Just before observation, 20 μM coelenterazine-h was added to the culture medium. To image the transient Ca 2+ induced by high-potassium stimulation, cells were treated with 50 mM KCl. Luminescence images were collected at 10 Hz. Preparation and imaging of D. discoideum Strain Ax-2 was cultured in HL-5 medium as previously described [27] . Expression plasmids were electroporated into cells, and transformants were selected in the presence of 10 μg ml −1 G418 (Life Technologies). For cAMP imaging, the cells were starved in development buffer (10 mM K/Na 2 phosphate buffer, 1 mM CaCl 2 and 2 mM MgCl 2 ; pH 6.5) for at least 6 h and were plated in 35-mm glass-bottom dishes or on 1% agar plates. The detailed imaging conditions are described in the Supplementary Methods and Supplementary Table S6 . Preparation and imaging of plants Wild-type and transformed Arabidopsis thaliana plants (ecotype Columbia, Col-0) were grown at 22 °C under 16 h light/dark. The Arabidopsis plants were transformed with pH2GW7_CT- Nano-lantern (ATP1) using Agrobacterium tumefaciens (strain GV3101) to generate stable transgenic plants. Transformants were selected on MS medium containing 20 μg ml −1 hygromycin B, and the T2 plants were used for imaging. Wild-type Nicotiana benthamiana plants were grown at 26 °C under 16-h light/dark. N. benthamiana plants were transfected with pH2GW7_Nano-lantern (ATP1) for transient expression by the agroinfiltration method and were imaged 1 day after agroinfiltration. To observe the effect of photosynthesis on ATP dynamics, we applied 438/24 nm blue light (LightEngine SPECTRA; Lumencor). Because visible light excitation causes strong chloroplast autofluorescence, we used the same instrumental and optical setup as described above for the Nano-lantern (Ca 2+ ) imaging induced by ChR2 stimulation to avoid perturbation of CT-Nano-lantern (ATP1) signals. The detailed imaging conditions are described in Supplementary Methods and Supplementary Table S6 . Accession codes: Sequences have been deposited in GenBank under the accession codes JN859492 (Nano-lantern), JN859493 (Nano-lantern (Ca 2+ ) CaM-2G), JN859494 (Nano-lantern (Ca 2+ ) CaM-2GS), JN859495 (Nano-lantern (Ca 2+ ) CaM-4GS), JN859496 (Nano-lantern (Ca 2+ ) CaM(E104Q)-2G), JN859497 (Nano-lantern (Ca 2+ ) CaM(E104Q)-3GS), JN859498 (Nano-lantern (Ca 2+ ) CaM(E104Q)-4GS), JN859499 (Nano-lantern (cAMP 0.4)), JN859500 (Nano-lantern (cAMP1.6)), JN859501 (Nano-lantern (cAMP 3.3), JN859502 (Nano-lantern (ATP1)), JN859503 (CT-Nano-lantern (ATP1)) and JN974906 (Nano-lantern (ATP0)). How to cite this article: Saito, K. et al. . Luminescent proteins for high-speed single-cell and whole-body imaging. Nat. Commun. 3:1262 doi: 10.1038/ncomms2248 (2012).